Experimental orthotopic transplantation of a tissue-engineered oesophagus in rats A tissue-engineered oesophageal scaffold could be very useful for the treatment of pediatric and adult patients with benign or malignant diseases such as carcinomas, trauma or congenital malformations. Here we decellularize rat oesophagi inside a perfusion bioreactor to create biocompatible biological rat scaffolds that mimic native architecture, resist mechanical stress and induce angiogenesis. Seeded allogeneic mesenchymal stromal cells spontaneously differentiate (proven by gene-, protein and functional evaluations) into epithelial- and muscle-like cells. The reseeded scaffolds are used to orthotopically replace the entire cervical oesophagus in immunocompetent rats. All animals survive the 14-day study period, with patent and functional grafts, and gain significantly more weight than sham-operated animals. Explanted grafts show regeneration of all the major cell and tissue components of the oesophagus including functional epithelium, muscle fibres, nerves and vasculature. We consider the presented tissue-engineered oesophageal scaffolds a significant step towards the clinical application of bioengineered oesophagi. Globally, every year, over 500,000 individuals are diagnosed with oesophageal cancer [1] , a figure predicted to increase to 850,000 by 2030 (ref. 2 ). About 30% of them [3] , as well as patients with traumatic and congenital disorders (occurring in 1:2,500 to 1:4,500 live births), ultimately have to undergo surgical resection of the oesophagus. A variety of surgical options are available to restore digestive continuity including substitutions using tissue conduits harvested from stomach [4] , colon or jejunum [5] . However, these reconstructive procedures are complex and are associated with substantial morbidity [6] and mortality [7] . Two years after oesophagectomy, many patients suffer from dysphagia and commonly need to undergo endoscopic interventions to dilate strictures [8] . For oesophageal atresia, even the mildest form has mediocre long-term functionality, 81% of operated children suffer from gastrointestinal symptoms (mainly dysphagia and reflux symptoms) several years after the surgery [9] . A tissue-engineering approach, where a transplantable conduit is bioengineered to replace the resected segment, thus eliminating the need to harvest replacement tissues form the patient’s own body, would avoid high-risk surgeries, be readily available and likely reduce the surgery-related mortality and morbidity and improve long-term functional outcome. Moreover, patients who today are considered inoperable because of poor clinical status could be given consideration. Tissue engineering usually includes a scaffold—that is, a three-dimensional (3D) structure for cells to adhere, proliferate and organize on. The scaffolds can be biologically derived or made from artificial materials (biodegradable or non-biodegradable). The scaffolds should exhibit several properties such as: (i) the ability to support cell growth, (ii) mechanical properties to withstand in vivo stress, (iii) angiogenesis induction and (iv) must be non-immunogenic (well tolerated by the recipient’s immune system). An oesophageal graft should be able to collapse while in a resting state and still be distensible to allow food bolus passage [10] , [11] . Once incorporated in the native tissue, the repopulated scaffold should ultimately be able to propagate peristalsis and withstand the low pH of gastric fluid. These properties are mediated by functional muscle layers and a mature epithelial layer. The regeneration of a functional external muscular layer is likely dependent on the extracellular matrix (ECM) that will direct the repopulating muscle cells. Previous clinical oesophageal tissue engineering attempts have focused on the application of extracellular matrices [12] or autologous oral mucosal cell sheets [13] to prevent postoperative stenosis after endoscopic removal of the mucosa and submucosa. Despite successful outcomes, a tissue-engineered replacement for full-wall segments of the oesophagus is still unattainable, as demonstrated by earlier preclinical regenerative attempts reporting stricture [14] , [15] , [16] , [17] , [18] , dilatation [14] , leakage [19] and fistula formation [15] . Decellularization is a process that reduces the immunogenicity of an organ or tissue by removing cellular elements while retaining mechanical and bioactive properties of the organ. The optimal decellularization method varies for each specific tissue/organ but generally includes application of reagents (such as detergents and enzymes) and/or physical methods (sonication, freeze/thaw, agitation and so on) [20] . Using these methods, biological scaffolds can be obtained for many organs such as hearts [21] , blood vessels [22] , lungs [23] , kidney [24] and livers [25] . Each of these decellularized scaffolds retain its organ-specific unique ECM composition [20] . On the basis of our previous preclinical and clinical experience with tissue-engineered airways [26] , [27] , [28] , we successfully develop and characterize an oesophageal scaffold and subsequently demonstrate its functional in vivo regenerative properties in an orthotopic rat model ( Fig. 1 ). 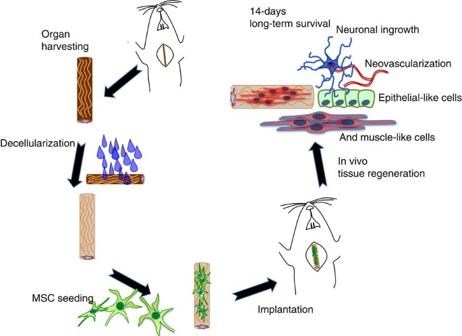Figure 1: Study overview. Donor oesophagi were decellularized and reseeded with bone marrow mesenchymal stromal cells. After 3-week culture, the grafts were used to replace the entire cervical oesophagus of the recipient animal. All animals survived until the 2-week time point, and further evaluations of the explanted grafts were performed. Figure 1: Study overview. Donor oesophagi were decellularized and reseeded with bone marrow mesenchymal stromal cells. After 3-week culture, the grafts were used to replace the entire cervical oesophagus of the recipient animal. All animals survived until the 2-week time point, and further evaluations of the explanted grafts were performed. Full size image Creation and characterization of oesophageal scaffold Oesophagi were harvested from adult Sprague–Dawley rats. We modified our airway decellularization protocol [26] to decellularize the organs in a submerged, luminal perfusion system. The reagents used were deoxycholate to disrupt cell membranes, deioniozed water to deliver an osmotic shock and DNase-I to digest nucleic acids. During the decellularization, the organ gradually turned translucent ( Fig. 2a–d ). The three distinct layers of the oesophagus—that is, mucosa, submucosa and external muscular layer—were identifiable and had a similar structure to that of the native organ but with the absence of cell nuclei ( Fig. 2e–h ). Masson’s trichrome staining revealed the retention of substantial amounts of collagen in similar configuration to the native organ ( Fig. 2i,j ). Elimination of intact cell nuclei was confirmed using 4′,6-diamidino-2-phenylindole (DAPI) ( Fig. 2k–m ). The perfusion method was proven to be superior to agitation systems, as agitation left many intact cell nuclei in the mucosa–submucosa ( Fig. 2l ). Computed tomography (CT) revealed a similar 3D structure in fresh (native; control) and decellularized organ ( Fig. 2n,o ). Scanning electron microscopy (SEM) of the external sides of the native and decellularized oesophagi showed similar presence of fibres ( Fig. 2p,q ). A computer-based evaluation further revealed a moderate decrease in fibre diameter by 40% and a highly preserved fibre orientation ( E =0.12±0.9 and E =0.15±0.9 for the native and decellularized oesophagus, respectively, n =3; Fig. 2r,s ). SEM of the luminal side of the native oesophagus demonstrated a scale-like appearance indicating the presence of cells, while the decellularized organ had a smooth, intact basement membrane ( Fig. 2t,u ). We evaluated macroscopic fibre orientation by tractography based on magnetic resonance imaging. Tracts were less abundant in the decellularized tissue, probably due to the loss of cells, but revealed similar orientations to native tissue ( Fig. 3 ). Using immunohistochemistry, several residual bioactive proteins such as elastin, fibronectin, laminin and collagen were identified in the decellularized oesophagi. It has been shown that varying concentrations of collagen in the ECM can induce different cell fates [29] . Collagen also affects substrate stiffness, which in turn has an impact on cell fate. Thus, maintaining the collagen expression in the scaffold is important for cell differentiation. The scaffold demonstrated similar expressions for collagen I and IV as compared with the native tissue ( Fig. 4a–d ). The function of the basement membrane is to allow selective permeability and provide integrity [30] . An intact basement membrane was observed in the scaffold using SEM ( Fig. 2u ) and confirmed by collagen IV staining ( Fig. 4d ). Elastin has an important role in chemotaxis, cell adhesion and proliferation as well as a unique ability to recoil [31] . The scaffold displayed no altered protein expression or morphological changes to the elastin with respect to the native tissue ( Fig. 4e,f ). Fibronectin and laminin are important for cell adhesion and migration; both were expressed in the matrix in a manner similar to the native tissue ( Fig. 4g–j ). Blood supply to the regenerated graft is necessary for supplying oxygen and removing cellular metabolites. Lack of neovascularization would result in cell death and graft ischemia. By elastin and vascular endothelial growth factor (VEGF) staining, intact vasculature was identified in the scaffold and in the native tissue ( Fig. 4i–l inserts). Quantification of ECM proteins revealed that the decrease in most cases was insignificant ( Fig. 4m ). To evaluate functional angiogenesis induction, the chorioallantoic membrane (CAM) assay was performed. Collagen sponges with either phosphate-buffered saline (PBS) or VEGF were used as negative and positive controls. Macroscopic observations of CAM treated with decellularized oesophagi showed that the samples induced a spoke-wheel-like pattern development of vessels, and new vessels were sometimes arranged in loops around samples suggesting that decellularized matrices positively affected the growth and organization of the network of CAM vessels ( Fig. 4n,o ). SEM micrographs confirmed that the samples were encircled by CAM vessels ( Fig. 4p,q ). The quantification of the vessels converging towards the implants proved that decellularized oesophageal matrices stimulated a significant increase in the number of blood vessels compared with negative controls ( Fig. 4r ), suggesting a pro-angiogenic effect of decellularized oesophageal matrices. 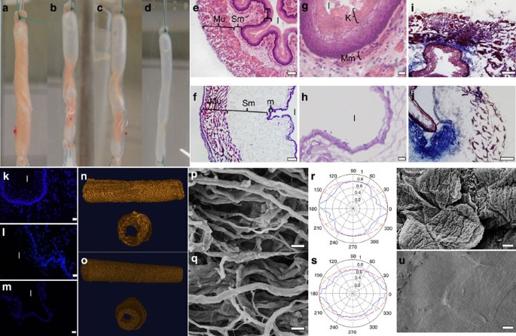Figure 2: Gross appearance and architectural evaluation of decellularized oesophagus. (a–d) Gross morphology of the oesophagus after perfusion decellularization process at 0 (a), 30 (b), 60 (c) and 120 min (d). (e–h) Haematoxylin and eosin staining showing mucosa (m), submucosa (sm), muscularis externa (mu) and lumen (l) in native (e,g) and decellularized (f,h) oesophagus (scale bar—100 μm). Higher magnification of the mucosa showing lumen (l), keratin (k) and muscularis mucosa (mm) of native oesophagus (g; scale bar—20 μm). No cell nuclei or keratin are visible in the mucosa of decellularized oesophagus, lumen is marked (l) (h). (i,j) Masson’s trichrome staining of native (i) and decellularized (j) oesophagus, showing the retention of collagen (blue) in the submucosa (scale bar—100 μm). (k–m) 4′,6-diamidino-2-phenylindole (DAPI) showing cell nuclei in a multilayered configuration close to the lumen (l) in native (k) and oesophagus decellularized using agitation (l) while in the perfusion group (m) the staining is weaker, smeared and without any intact cell nuclei (scale bar—50 μm). (n,o)Micro CT scan of native (n) and decellularized (o) oesophagus. (p–u) SEM evaluations of external side of native (p) and decellularized (q) oesophagus (scale bar—5 μm). Computer-based fibre evaluation showing the similarity of orientation between native (r) and decellularized oesophagus (s), blue line: computed pattern representative of fibre orientation. Red line: fitting ellipse of the computed pattern. SEM of luminal surface of the native oesophagus with flattened, cuboidal epithelial cells (t) and decellularized oesophagus showing a smooth basement membrane (u; scale bar—4 μm). Figure 2: Gross appearance and architectural evaluation of decellularized oesophagus. ( a – d ) Gross morphology of the oesophagus after perfusion decellularization process at 0 ( a ), 30 ( b ), 60 ( c ) and 120 min ( d ). ( e – h ) Haematoxylin and eosin staining showing mucosa (m), submucosa (sm), muscularis externa (mu) and lumen (l) in native ( e , g ) and decellularized ( f , h ) oesophagus (scale bar—100 μm). Higher magnification of the mucosa showing lumen (l), keratin (k) and muscularis mucosa (mm) of native oesophagus ( g ; scale bar—20 μm). No cell nuclei or keratin are visible in the mucosa of decellularized oesophagus, lumen is marked (l) ( h ). ( i , j ) Masson’s trichrome staining of native ( i ) and decellularized ( j ) oesophagus, showing the retention of collagen (blue) in the submucosa (scale bar—100 μm). ( k – m ) 4′,6-diamidino-2-phenylindole (DAPI) showing cell nuclei in a multilayered configuration close to the lumen (l) in native ( k ) and oesophagus decellularized using agitation ( l ) while in the perfusion group ( m ) the staining is weaker, smeared and without any intact cell nuclei (scale bar—50 μm). ( n , o )Micro CT scan of native ( n ) and decellularized ( o ) oesophagus. ( p – u ) SEM evaluations of external side of native ( p ) and decellularized ( q ) oesophagus (scale bar—5 μm). Computer-based fibre evaluation showing the similarity of orientation between native ( r ) and decellularized oesophagus ( s ), blue line: computed pattern representative of fibre orientation. Red line: fitting ellipse of the computed pattern. SEM of luminal surface of the native oesophagus with flattened, cuboidal epithelial cells ( t ) and decellularized oesophagus showing a smooth basement membrane ( u ; scale bar—4 μm). 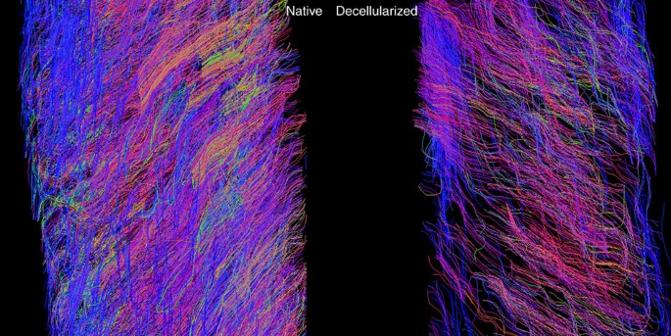Figure 3: Tractography evaluation. Tractography based on diffusion tensor imaging of native (left) and decellularized (right) rat oesophagus. The general fibre orientations are maintained but fewer tracts were detected in the decellularized sample. Full size image Figure 3: Tractography evaluation. Tractography based on diffusion tensor imaging of native (left) and decellularized (right) rat oesophagus. The general fibre orientations are maintained but fewer tracts were detected in the decellularized sample. 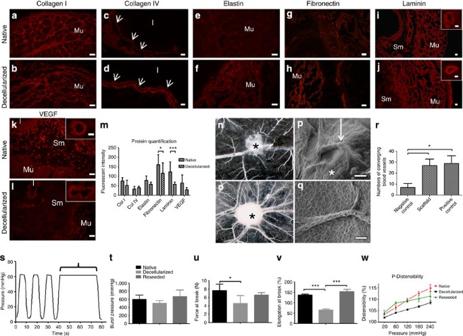Figure 4: Protein content and functional assays. (a–d) Expression of collagen I and IV in native (a,c) and decellularized (b,d) oesophagus (scale bar—Col I—50 μm, Col IV—20 μm, mu indicating muscular layer, l—lumen). An intact basement membrane is indicated by collagen IV expression (c,d, red arrows). (e–j) Expression of elastin, fibronectin and laminin in native (e,g,i, mu indicating muscular layer, sm submucosa) and decellularized (f,h,j) oesophagus (scale bar—25 μm). (k,l) Expression of VEGF factor in native (k) and decellularized (l) oesophagus (l—lumen, sm—submucosa, mu—muscular layer). VEGF and laminin-stained tubular structures, suggesting intact vasculature, are found in native and decellularized tissue (i–l, inserts, scale bar—10 μm). (m) Protein quantification of extracellular matrix proteins (n=3 biological replicates). (n–q) Angiogenesis assay implanted with gelfoam (control, asterisk inn) and with fragments of decellularized oesophagus (asterisk ino). The oesophagus induced new vessels, proving the scaffolds’ positive influence of vessel organization. SEM micrographs of vessel and the scaffold sample (p, *) and newly built vessel (p, ↓) (scale bar—100 μm), higher magnification on one of the vessels(q; scale bar—25 μm). (r) Quantification of blood vessels converging to the samples, indicating the strong angiogenic induction by the scaffold, at the levels of the positive control (n=3). (s) The scaffold was inflated and deflated over 10,000 times, a stable plateau phase (s) proves the scaffold’s integrity in the last cycle, as there is no leakage from the scaffold (n=3, one representative graph shown). (t) Axial strength was evaluated using burst pressure measurements, without any difference between native, decellularized or reseeded groups (n=5). (u,v) Tensile test showed that strength lost during decellularization was regained after reseeding: force at break (u) and strain at break (v) (n=5). (w) Distensibility assay showed that the lost distensibility after decellularization (black series) was regained after reseeding (green series) (n=5), highly resembling the native organ (red series). *P<0.05, ***P<0.001 by analysis of variance (ANOVA) followed by Tukey’spost hoctests for (r,u,v), or ANOVA followed by Bonferroni post tests for (m,w). Full size image Figure 4: Protein content and functional assays. ( a – d ) Expression of collagen I and IV in native ( a , c ) and decellularized ( b , d ) oesophagus (scale bar—Col I—50 μm, Col IV—20 μm, mu indicating muscular layer, l—lumen). An intact basement membrane is indicated by collagen IV expression ( c , d , red arrows). ( e – j ) Expression of elastin, fibronectin and laminin in native ( e , g , i , mu indicating muscular layer, sm submucosa) and decellularized ( f , h , j ) oesophagus (scale bar—25 μm). ( k , l ) Expression of VEGF factor in native ( k ) and decellularized ( l ) oesophagus (l—lumen, sm—submucosa, mu—muscular layer). VEGF and laminin-stained tubular structures, suggesting intact vasculature, are found in native and decellularized tissue ( i – l , inserts, scale bar—10 μm). ( m ) Protein quantification of extracellular matrix proteins ( n =3 biological replicates). ( n – q ) Angiogenesis assay implanted with gelfoam (control, asterisk in n ) and with fragments of decellularized oesophagus (asterisk in o ). The oesophagus induced new vessels, proving the scaffolds’ positive influence of vessel organization. SEM micrographs of vessel and the scaffold sample ( p , *) and newly built vessel ( p , ↓) (scale bar—100 μm), higher magnification on one of the vessels( q ; scale bar—25 μm). ( r ) Quantification of blood vessels converging to the samples, indicating the strong angiogenic induction by the scaffold, at the levels of the positive control ( n =3). ( s ) The scaffold was inflated and deflated over 10,000 times, a stable plateau phase ( s ) proves the scaffold’s integrity in the last cycle, as there is no leakage from the scaffold ( n =3, one representative graph shown). ( t ) Axial strength was evaluated using burst pressure measurements, without any difference between native, decellularized or reseeded groups ( n =5). ( u , v ) Tensile test showed that strength lost during decellularization was regained after reseeding: force at break ( u ) and strain at break ( v ) ( n =5). ( w ) Distensibility assay showed that the lost distensibility after decellularization (black series) was regained after reseeding (green series) ( n =5), highly resembling the native organ (red series). * P <0.05, *** P <0.001 by analysis of variance (ANOVA) followed by Tukey’s post hoc tests for ( r , u , v ), or ANOVA followed by Bonferroni post tests for ( m , w ). Full size image The correct biomechanical properties are pivotal for successful clinical outcomes. A stress test involving repeated injection and withdrawal of air into the scaffold was applied for 72 h. After more than 10,000 cycles, the integrity of the scaffold was still maintained, as proven by the absence of leakage ( Fig. 4s ). The burst pressure was determined by injecting air until the point of burst in segments of native, decellularized and reseeded oesophagi. No significant difference between the three groups was observed ( Fig. 4t ). To evaluate longitudinal biomechanical properties, native, decellularized and reseeded segments of oesophagi were elongated until rupture. The decellularization partly compromised the biomechanical properties of the organ, but the strength was regained after reseeding ( Fig. 4u,v ). Organ distensibility was evaluated in native, decellularized and reseeded organs by assessing pressure-diameter relationship. The organs were exposed to incremental steps of intraluminal pressure and the changes in external diameter were assessed using a digital image acquisition. The studies revealed that the decellularized organ was less distensible than native. However, the distensibility of the reseeded organ closely resembled the native ( Fig. 4w ), further strengthening the evidence for biomechanical recovery in reseeded organ. Immunogenicity of the decellularized scaffold In vivo immune responses were evaluated by subcutaneous transplantations into allogeneic rats. Three groups were used: decellularized scaffold, native organ and sham surgery. After 5 days, the native organ was heavily damaged and infiltrated by inflammatory cells ( Fig. 5a ). In contrast, the decellularized organ was intact ( Fig. 5b ), the muscular layer remained undamaged and cell infiltration in surrounding tissue was similar to that of the sham group ( Fig. 5c ). Macrophages are important for host response to grafts [32] , [33] and wound healing [34] . Macrophage quantification revealed that the transplanted native oesophagus induced a significant increase in macrophage recruitment when compared with both decellularized graft and sham group. There were no differences in macrophage numbers between decellularized graft and sham group. These results suggest that the graft was well tolerated by the recipient and did not induce adverse immune responses ( Fig. 5d–g ). A considerable reduction of DNA was observed after decellularization ( Fig. 5h ). Staining for major histocompatibility complexes (MHCs) I and II, essential for the foreign body response, revealed the complete absence of positive cells in the decellularized oesophagi ( Fig. 5i–l ). 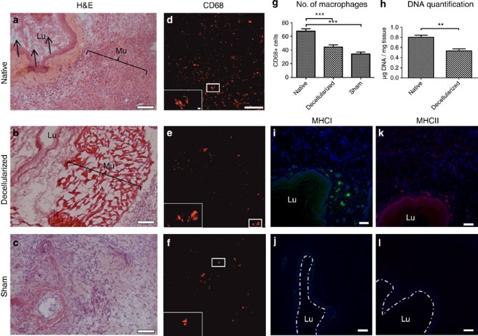Figure 5: Immunogenic properties of the scaffold. (a–c) Histology from 5-day subcutaneous transplantations of native, decellularized oesophagi and sham surgery (scale bar—100 μm). The native organ was heavily infiltrated with host cells resulting in almost complete destruction of the graft. The muscular layer shows almost total degradation (a, bracket) and the lumen (a, lu) has been invaded by cells (a, arrowhead). In contrast, the decellularized organ has an intact muscular layer (b, bracket) and fewer infiltrating cells. The scaffold’s integrity also appeared intact as no cells were invading to the lumen (b, lu marks lumen, mu muscular layer). The sham surgery (c) showed similar inflammatory response as the decellularized group. (d–f) Macrophages in the subcutaneous implantation groups were stained and quantified. There was a considerable increase in CD68 positive cells in the native, allotransplantation (d) as compared with both decellularized organ (e) and sham surgery groups (skin incision) (f) (scale bar—67 μm, insert scale bars—11 μm). (g) Quantification of number of macrophages in each group, showed differences between native group and the other two, but no difference between decellularized oesophagus and sham groups (n=3). (h) The DNA content in the decellularized organ was moderately decreased compared with the native organ. (i–l) Major histocompatibility complexes I- and II-positive cells were totally eliminated in decellularized oesophagus (j,l) compared with native oesophagus (i,k) (scale bar—50 μm). ***P<0.001 by ANOVA followed by Tukey’spost hoctests for (g). **P<0.001 by Student’st-test for (h). Figure 5: Immunogenic properties of the scaffold. ( a – c ) Histology from 5-day subcutaneous transplantations of native, decellularized oesophagi and sham surgery (scale bar—100 μm). The native organ was heavily infiltrated with host cells resulting in almost complete destruction of the graft. The muscular layer shows almost total degradation ( a , bracket) and the lumen ( a , lu) has been invaded by cells ( a , arrowhead). In contrast, the decellularized organ has an intact muscular layer ( b , bracket) and fewer infiltrating cells. The scaffold’s integrity also appeared intact as no cells were invading to the lumen ( b , lu marks lumen, mu muscular layer). The sham surgery ( c ) showed similar inflammatory response as the decellularized group. ( d – f ) Macrophages in the subcutaneous implantation groups were stained and quantified. There was a considerable increase in CD68 positive cells in the native, allotransplantation ( d ) as compared with both decellularized organ ( e ) and sham surgery groups (skin incision) ( f ) (scale bar—67 μm, insert scale bars—11 μm). ( g ) Quantification of number of macrophages in each group, showed differences between native group and the other two, but no difference between decellularized oesophagus and sham groups ( n =3). ( h ) The DNA content in the decellularized organ was moderately decreased compared with the native organ. ( i – l ) Major histocompatibility complexes I- and II-positive cells were totally eliminated in decellularized oesophagus ( j , l ) compared with native oesophagus ( i , k ) (scale bar—50 μm). *** P <0.001 by ANOVA followed by Tukey’s post hoc tests for ( g ). ** P <0.001 by Student’s t -test for ( h ). Full size image Adhesion and differentiation of seeded MSCs The in vivo outcome of transplanted tracheal scaffolds has been shown to depend on cells seeded to both luminal and external surfaces [35] . We isolated bone marrow mesenchymal stromal cells (BM-MSCs) based on their plastic adherence properties and characterized them using flow cytometry according to our previous study [36] . To evaluate the decellularized oesophagus’ cytocompatibility, green-fluorescent protein (GFP)-transfected MSCs were seeded on either the epithelial or muscular surface of the organ and allowed to adhere. Interestingly, we found that after the initial 48 h, different characteristics on each side of the scaffold considerably affected cell morphology, with more elongated cells on the muscular side ( Fig. 6a,b ), compared with more cuboidal cells on the epithelial side ( Fig. 6d,e ). On both sides, cells positive for the proliferation marker Ki-67 were detected ( Fig. 6c,f ). These specific morphologies were retained after 3-week culture, after which the cells also stained positively for epithelial (pankeratin, tight junction protein zona occludens 2) and muscular markers (MyoD1, desmin; Fig. 6g–l ).The seeded cells were proven to be metabolically active by 3-(4,5-dimethylthiazol-2-yl)-2,5-diphenyltetrazolium bromide assay ( Fig. 6m ). Cells cultured for 3 weeks on either plastic, muscular side or epithelial side of the scaffold were evaluated for gene expression. All three groups retained the MSC-marker CD90 . Cells grown on the muscular side showed a small but significant increase in desmin , while cells grown on the epithelial side showed upregulation of the epithelial differentiation gene SP1 ( Fig. 6n ). The following genes relevant for epithelial and muscular differentiation were not detected in either of the groups: KRT5, KRT10, KRT14, Myf6 and Myog . We further tested the cells grown on the scaffold functionally. We found that the cells grown on the scaffold for 3 weeks, but not cells grown on plastic, exhibited calcium influxes in response to high extracellular potassium ions ( Fig. 6o ). This suggests that cells that had been in contact with the scaffold acquired an excitable phenotype, likely by the expression of voltage-dependent ion channels. Electrical resistance is commonly used to measure the health and function of epithelial cells grown in culture dish inserts [37] . We created a custom construct for mounting the scaffold and measured the resistance before and after reseeding and found a small, but significant, increase in resistance, suggesting a functional epithelial barrier ( Fig. 6p ). 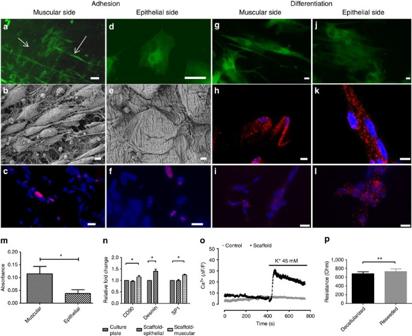Figure 6: Cell-scaffold interaction. (a) GFP-positive cells on the muscular side of the scaffold showed an elongated morphology 48 h after seeding, with cells aligned in two main orientations (arrows), which corresponded to the directions of muscular layer’s fibres (scale bar—50 μm). (b) SEM image confirmed cell morphology (scale bar—5 μm). (c) Ki-67 (red) proved the presence of proliferative cells on scaffold (nuclei counterstained with DAPI, scale bar—50 μm). (d,e) Cells seeded to the epithelial side of the scaffold had a cuboidal shape (d, green—GFP, scale bar—50 μm), further confirmed by SEM (e, scale bar—5 μm). (f) Ki-67 showed the presence of proliferative cells on the epithelial layer (scale bar—50 μm). (g–i) After 3-week culture, the cells on the muscular side retained the elongated morphology (g) and stained positive for muscular markers myoD1 (h) and desmin (i) (green—GFP, markers red, nuclei stain DAPI (blue) scale bar—10 μm). (j–l) Cells grown on the epithelial side for 3 weeks showed cuboidal morphology and were positive for epithelial markers pan-keratin (k) and tight junction protein zona occludens-2 (l) (green—GFP, markers red, nuclei-stained DAPI (blue) scale bar—10 μm). (m) 3-(4,5-dimethylthiazol-2-yl)-2,5-diphenyltetrazolium bromide assay proved that the cells were metabolically active on the scaffold (n=3). (n) qPCR showed that the cells retained their MSC markerCD90but had different gene expression for muscular (desmin) and epithelial (sp1) differentiation markers depending on location of growth (n=3). (o) Cells grown on either culture plates or cryosections of the decellularized scaffolds for 3 weeks were loaded with a calcium dye and tested for calcium fluxation. Elevation of extracellular K+ concentration triggered calcium transients only in cells grown on the scaffold in contrast to the cells grown on culture dish (control). (p) The decellularized mucosa’s electrical resistance showed a small but significant increase after reseeding and culturing for 3 weeks (n=3). *P<0.05 by ANOVA followed by Tukey’spost hoctests for (n). *P<0.05, **P<0.01 by unpaired (m) and paired (p) Student’st-test. Figure 6: Cell-scaffold interaction. ( a ) GFP-positive cells on the muscular side of the scaffold showed an elongated morphology 48 h after seeding, with cells aligned in two main orientations (arrows), which corresponded to the directions of muscular layer’s fibres (scale bar—50 μm). ( b ) SEM image confirmed cell morphology (scale bar—5 μm). ( c ) Ki-67 (red) proved the presence of proliferative cells on scaffold (nuclei counterstained with DAPI, scale bar—50 μm). ( d , e ) Cells seeded to the epithelial side of the scaffold had a cuboidal shape ( d , green—GFP, scale bar—50 μm), further confirmed by SEM ( e , scale bar—5 μm). ( f ) Ki-67 showed the presence of proliferative cells on the epithelial layer (scale bar—50 μm). ( g – i ) After 3-week culture, the cells on the muscular side retained the elongated morphology ( g ) and stained positive for muscular markers myoD1 ( h ) and desmin ( i ) (green—GFP, markers red, nuclei stain DAPI (blue) scale bar—10 μm). ( j – l ) Cells grown on the epithelial side for 3 weeks showed cuboidal morphology and were positive for epithelial markers pan-keratin ( k ) and tight junction protein zona occludens-2 ( l ) (green—GFP, markers red, nuclei-stained DAPI (blue) scale bar—10 μm). ( m ) 3-(4,5-dimethylthiazol-2-yl)-2,5-diphenyltetrazolium bromide assay proved that the cells were metabolically active on the scaffold ( n =3). ( n ) qPCR showed that the cells retained their MSC marker CD90 but had different gene expression for muscular ( desmin ) and epithelial ( sp1 ) differentiation markers depending on location of growth ( n =3). ( o ) Cells grown on either culture plates or cryosections of the decellularized scaffolds for 3 weeks were loaded with a calcium dye and tested for calcium fluxation. Elevation of extracellular K+ concentration triggered calcium transients only in cells grown on the scaffold in contrast to the cells grown on culture dish (control). ( p ) The decellularized mucosa’s electrical resistance showed a small but significant increase after reseeding and culturing for 3 weeks ( n =3). * P <0.05 by ANOVA followed by Tukey’s post hoc tests for ( n ). * P <0.05, ** P <0.01 by unpaired ( m ) and paired ( p ) Student’s t -test. Full size image Orthotopic transplantation of oesophageal grafts Before orthotopic transplantation, a 4-cm long decellularized oesophagus was seeded with rat BM-MSCs and maintained in culture for 3 weeks. Cell attachment to the graft was confirmed by imaging of GFP-positive cells using a fluorescent microscope ( Fig. 7a ). Fifteen-millimetre-long segments, corresponding to 20% of the total length, were used for orthotopic transplantation. Under general anaesthesia, the recipient’s trachea and oesophagus were exposed through an anterior midline cervical incision. The trachea was partly opened to facilitate breathing during the operation. As control, a sham surgery was performed by resecting a 15-mm segment of the oesophagus, and re-anastomozing it using the same anastomotic technique detailed below. A 15-mm segment of the oesophagus was removed and replaced with the engineered graft ( Fig. 7b ) using 7-0 monofilament-interrupted sutures with knots tied extraluminally. During the postoperative period, the animals were fed a liquid diet for 7 days, after which a soft food diet was provided for the remaining 7 days. The animals, although initially immobile, quickly recovered and did not show any significant signs of pain or health impairment according to a pain assessment scale [38] and general health scale ( Supplementary Movie 1 ). Interestingly, the transplanted animals’ weight curves were significantly better than those of the sham surgery group from day 4 onward ( Fig. 7c ). 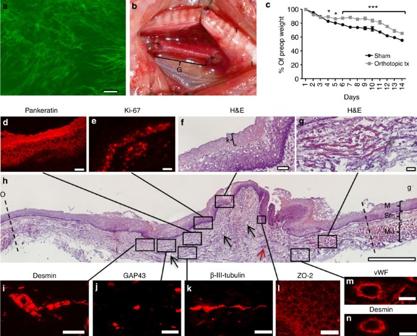Figure 7: Fourteen-day orthotopic transplantation. (a) GFP-positive cells after 3 weeks’ culture on tubular scaffold (scale bar—50 μm). (b) Orthotopic replacement of the entire cervical oesophagus with a reseeded tissue-engineered graft (g), the trachea (t) was partially opened (*) to facilitate breathing, the lower part of the larynx is observed (l). (c) Postoperative weight curves. The animals receiving tissue-engineered grafts lost weight in lesser extent to control surgery and weight gain was observed at some time points (* indicate significance levels between the groups). (d) The neo-epithelium stained positively for pankeratin (scale bar—50 μm). (e) Proliferative cells were found in the basal part of the epithelium (scale bar—20 μm). (f) High power magnification showed a seven- to nine-layer thick epithelium with a superficial keratin layer (f, k; scale bar—50 μm). (g) High power magnification of regenerated muscle fibres (scale bar—50 μm). (h) Sagittal section of the oesophageal wall, the whole graft (marked with dashed lines) was re-epithelized, several blood vessels (black arrows), a few accumulations of inflammatory cells (red arrow) were found. (scale bar—500 μm. m indicates mucosa, sm submucosa, mu muscular layer, o and g indicate oral and gastric sides of the explant). (i–n) Repopulation of the scaffold of different cell types was proven by immunohistochemistry (scale bars—50 μm, for ZO 2–20 μm); desmin-positive cells were found throughout the graft (i), Gap43 and Beta-III-tubulin-positive staining suggested in-growth of neurons (j,k). Zona occludens-II, a tight junction protein, showed a pattern consistent with a healthy epithelium (l). Potential vasculature stained positively for von willebrand factor (m) out of which some stained positively for desmin (n), suggesting arterioles. *P<0.05, ***P<0.001 by ANOVA followed by Bonferroni post tests for (c). Figure 7: Fourteen-day orthotopic transplantation. ( a ) GFP-positive cells after 3 weeks’ culture on tubular scaffold (scale bar—50 μm). ( b ) Orthotopic replacement of the entire cervical oesophagus with a reseeded tissue-engineered graft (g), the trachea (t) was partially opened (*) to facilitate breathing, the lower part of the larynx is observed (l). ( c ) Postoperative weight curves. The animals receiving tissue-engineered grafts lost weight in lesser extent to control surgery and weight gain was observed at some time points (* indicate significance levels between the groups). ( d ) The neo-epithelium stained positively for pankeratin (scale bar—50 μm). ( e ) Proliferative cells were found in the basal part of the epithelium (scale bar—20 μm). ( f ) High power magnification showed a seven- to nine-layer thick epithelium with a superficial keratin layer ( f , k; scale bar—50 μm). ( g ) High power magnification of regenerated muscle fibres (scale bar—50 μm). ( h ) Sagittal section of the oesophageal wall, the whole graft (marked with dashed lines) was re-epithelized, several blood vessels (black arrows), a few accumulations of inflammatory cells (red arrow) were found. (scale bar—500 μm. m indicates mucosa, sm submucosa, mu muscular layer, o and g indicate oral and gastric sides of the explant). ( i – n ) Repopulation of the scaffold of different cell types was proven by immunohistochemistry (scale bars—50 μm, for ZO 2–20 μm); desmin-positive cells were found throughout the graft ( i ), Gap43 and Beta-III-tubulin-positive staining suggested in-growth of neurons ( j , k ). Zona occludens-II, a tight junction protein, showed a pattern consistent with a healthy epithelium ( l ). Potential vasculature stained positively for von willebrand factor ( m ) out of which some stained positively for desmin ( n ), suggesting arterioles. * P <0.05, *** P <0.001 by ANOVA followed by Bonferroni post tests for ( c ). Full size image Histological and functional graft evaluation post mortem All animals survived to the study end point of 14 days and visual inspection showed patency of all oesophageal grafts. Hair, originating from the animals’ grooming, was frequently found in the graft. The oesophagus, longitudinally dissected, revealed a neo-mucosa covering the entire graft ( Fig. 7h ). Percentage of patency of the explanted grafts was assessed as previously described [39] and expressed as a ratio between graft diameter and adjacent native oesophagus. Mild reduction of patency was observed, but without statistical significance (71.50±11.65% SEM, n =10). Haematoxylin and eosin (H&E) staining revealed a stratified squamous neo-epithelium covering the full length of the graft, largely comparable to the native epithelium with basal cuboidal and suprabasal flattened cells. The number of cell layers and cell morphology of the graft were nearly identical to that of the native oesophageal epithelium. The harvested graft also showed a thick keratin layer ( Fig. 7f ) and there were no signs of organ rejection or adverse immunological responses [39] . Additionally, several newly developed blood vessels ( Fig. 7h ) and muscle fibres ( Fig. 7g ) were found in the graft. No GFP-positive cells were identified in the explanted grafts. Evaluation of the harvested graft showed pan-keratin expression throughout the internal surface of the graft ( Fig. 7d ), with proliferative basal cells ( Fig. 7e ) and aligned, elongated desmin-positive cells that indicates regeneration of the muscular layer ( Fig. 7i ). Positive immunohistochemistry staining for growth-associated protein 43 (Gap-43), an axonal regeneration marker [40] ( Fig. 7j ) and fibre-like orientation of Beta-III-tubulin (exclusively expressed in neurons; Fig. 7k ) on both sides of the graft indicated initial evidence for re-innervation and ongoing neo-neurogenesis. On H&E-stained sections, blood vessels could be detected ( Fig. 7h ) with positive von Willebrand factor staining indicated their endothelialization ( Fig. 7m ), some of which had a muscular component (artery/arterioli; Fig. 7n ). Contrast enhanced CT-scanning demonstrated a patent oesophagus with a smooth internal surface ( Fig. 8a ). By SEM, epithelial cells with regular folds and small intercellular spaces, suggesting a healthy epithelium, were detected in the explanted tissue ( Fig. 8b,c ). Using transmission electron microscopy (TEM) we observed a multilayered keratinized epithelium with rounded basal cells that matured towards the lumen with more stretched out morphology and smaller cell nuclei. As expected, bacteria were seen on the luminal surface of the oesophagus graft but none were found inside the tissue, confirming the integrity and barrier function of the neo-epithelium ( Fig. 8d ). Beneath the epithelium, a continuous basement membrane with underlying collagen fibres was observed ( Fig. 8e ). We identified muscle cells with detectable mitochondriae (M), sarcomeres (S) and z-lines (Z) in the deeper layers of the graft ( Fig. 8f ). 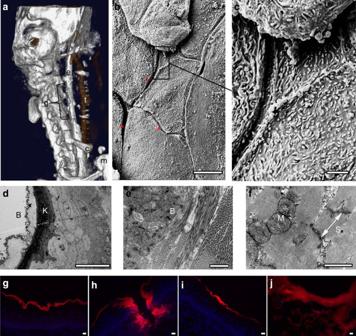Figure 8: Imaging and functional assays ofin vivoregenerated scaffold. (a) Contrast-enhanced computed tomography showed a smooth and patent oesophagus (bracket), anatomical landmarks: e—oesophagus, t—trachea (air-filled), c—clavicle, m—manubrium. (b,c) SEM of neo-epithelium showed a confluent cell layer with characteristic leaf-like morphology and small intercellular spaces (b, *) (scale bar—10 μm). Higher magnification of epithelial cells showed many folds in the cell membrane indicating a healthy epithelium (c; scale bar—2 μm). (d–f) TEM imaging showed a six- to eight-layered keratinized (d, K) epithelium with bacteria (d, B) only on the luminal side (d, B) (scale bar—10 μm). Aligned collagen fibres were seen underlying the basal membrane (e, B) (scale bar—1 μm). Deeper, muscle bundles were present, with abundant mitochondriae (f, M) and sarcomeres (f, S) bordered by Z-lines (f, Z) (scale bar—1 μm). (g–j) Biotin assay was performed to functionally test the regenerated epithelium. In the native epithelium, the staining was limited to the superficial surface (g), while a mechanically damaged epithelium showed a diffuse staining deeper in the epithelium (h). The regenerated epithelium (i) showed similar staining to the native epithelium. Assay performed on the decellularized scaffold showed a general diffusion through the mucosa to the submucosal (j; scale bar—20 μm). Figure 8: Imaging and functional assays of in vivo regenerated scaffold. ( a ) Contrast-enhanced computed tomography showed a smooth and patent oesophagus (bracket), anatomical landmarks: e—oesophagus, t—trachea (air-filled), c—clavicle, m—manubrium. ( b , c ) SEM of neo-epithelium showed a confluent cell layer with characteristic leaf-like morphology and small intercellular spaces ( b , *) (scale bar—10 μm). Higher magnification of epithelial cells showed many folds in the cell membrane indicating a healthy epithelium ( c ; scale bar—2 μm). ( d – f ) TEM imaging showed a six- to eight-layered keratinized ( d , K) epithelium with bacteria ( d , B) only on the luminal side ( d , B) (scale bar—10 μm). Aligned collagen fibres were seen underlying the basal membrane ( e , B) (scale bar—1 μm). Deeper, muscle bundles were present, with abundant mitochondriae ( f , M) and sarcomeres ( f , S) bordered by Z-lines ( f , Z) (scale bar—1 μm). ( g – j ) Biotin assay was performed to functionally test the regenerated epithelium. In the native epithelium, the staining was limited to the superficial surface ( g ), while a mechanically damaged epithelium showed a diffuse staining deeper in the epithelium ( h ). The regenerated epithelium ( i ) showed similar staining to the native epithelium. Assay performed on the decellularized scaffold showed a general diffusion through the mucosa to the submucosal ( j ; scale bar—20 μm). Full size image Biotin assay has been previously described as an epithelial functional evaluation [41] , [42] , [43] . Biotin does not penetrate through healthy epithelium due to cross-linking of tight junction proteins [43] . We used a native oesophagus as a positive control and found the staining limited to the superficial epithelial layer ( Fig. 8g ). A scalpel blade-damaged epithelium served as a control, and the staining was found to diffuse deeper into the epithelium ( Fig. 8h ). The in vivo regenerated epithelium ( Fig. 8i ) was remarkably similar to the positive control, while the staining had diffused into the submucosa of the decellularized scaffold ( Fig. 8j ). Larger images of nucleic acid staining are provided ( Fig. 9a,b ), as well as secondary only staining ( Fig. 9c ) and construct to measure epithelial resistance ( Fig. 9d ). 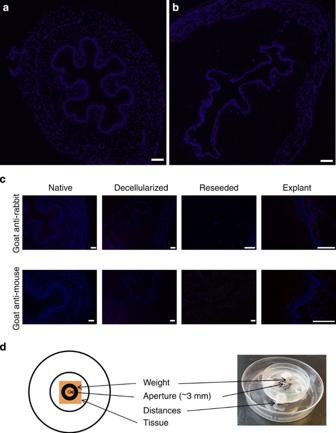Figure 9: Control staining and tissue electrical resistance construct. (a,b) Larger images of nuclear staining showed intact cell nuclei in the native oesophagus (a), while the decellularized oesophagus showed a smeared staining, without any intact cell nuclei (b, the intensity of the decellularized sample has been increased to easier identify the localization staining; scale bar—200 μm). (c) Secondary only staining of each representative antibody (scale bar—100 μm). (d) Custom-made construct to mount the tissue for electrical resistance testing. The tissue was separating the PBS in the two different Petri dishes and the electrical resistance between the two dishes was measured. Figure 9: Control staining and tissue electrical resistance construct. ( a , b ) Larger images of nuclear staining showed intact cell nuclei in the native oesophagus ( a ), while the decellularized oesophagus showed a smeared staining, without any intact cell nuclei ( b , the intensity of the decellularized sample has been increased to easier identify the localization staining; scale bar—200 μm). ( c ) Secondary only staining of each representative antibody (scale bar—100 μm). ( d ) Custom-made construct to mount the tissue for electrical resistance testing. The tissue was separating the PBS in the two different Petri dishes and the electrical resistance between the two dishes was measured. Full size image Despite many attempts to create a tissue-engineered graft to replace oesophageal tissue, no functional solution currently exists. The results from this study provide an important step forward towards the development of clinically successful tissue-engineered oesophageal replacements. With our perfusion protocol, we eliminated immunogenic properties from the oesophagus while preserving the critical components essential for a transplantable graft. We have drastically reduced the time required for decellularization, and have maintained the axial strength of the native tissue as compared with a previously described protocol using agitation [44] . The accelerated rate of decellularization by use of perfusion as compared with agitation may be explained by: (1) the resting state of the oesophagus is closed; therefore, under agitation the reagents act primarily upon the external esophagus, whereas perfusion opens the oesophagus and exposes the lumen to reagents, and (2) the application of hydrostatic pressure allows a greater penetration of the perfusate into the tissues [45] . The nanotopography of tissue-engineered scaffolds is crucial for adhesion, proliferation and differentiation of the seeded cells [46] , strongly suggesting the need to maintain the natural architecture in the decellularized tissue. The results indicate that our biological scaffold has similar histological architecture and molecular composition of collagen, fibronectin, elastin and laminin. Evaluations using SEM and tractography of the ECM fibres demonstrated that the structure of the native oesophagus is preserved after decellularization. DTI-based tractography has been used extensively in the field of neuroimaging to trace white matter tracts. On the basis of the diffusion direction of water molecules, an algorithm propagates tracts in the direction where the restriction of diffusion is low [47] . The same algorithms have also been applied to delineate the orientation of muscle fibres. This approach has been validated and shows good repeatability [48] . There are, however, limitations with the tractography used in the current study. First, parameters are adapted to the current data set, which makes analysis user-dependent. Second, tractography is ideally applied to isotropic voxel sizes. Anisotropic voxels used in the current study will favour tracts in the direction of the longest voxel dimension. However, the tractographies in the current study provide a biologically plausible result and offer a more macroscopic, but less detailed, visualization of the 3D structure in the decellularized oesophagus compared with the histological analysis. The similarity of the results between the native and decellularized oesophagi supports the validity of the analysis. Besides the preserved structural properties of the decellularized scaffold, the immunogenic profile of the graft plays a key role for successful implantation in vivo . The consensus is that DNA removal is crucial for avoiding adverse immune reaction; therefore, DNA quantification was used in this study to quantify the extent of decellularization. Several studies suggest a strong correlation between residual DNA and adverse host response [49] , [50] ; therefore DNA-based criteria were developed [51] . While attempting to reach adequately low levels of remaining DNA using a vigorous decellularization treatment, we observed extensive damage to the architecture of the ECM. Other studies have also reported that the mechanical properties [27] and the preservation of collagen and elastin [52] are compromised using extensive decellularization. More recent studies have considered the relationship between residual DNA and host response [51] . MHCs I and II have been clinically accepted to be relevant for acceptance of organ transplantations and the human equivalent, human leucocyte antigen, is routinely evaluated for acceptance of donor organ to the recipient [53] . As our scaffold contained no MHC I- or II-positive cells, we pursued an in vivo evaluation consisting of an implantation of the decellularized scaffold into subcutaneous tissue for 5 days, and compared this with the implantation of allogeneic scaffolds at the same site. Our results indicated that the scaffold was non-immunogenic while the allotransplanted oesophagus (native oesophagus) was (a) heavily infiltrated by inflammatory cells, (b) showed remarkable degradation of the muscular layer and (c) had cell infiltration into the lumen, indicating loss of integrity. In contrast to the allotransplantated graft, the decellularized scaffold was virtually intact, had few invading cells and preserved its integrity. Macrophages are one of the most important cells in the foreign body response and our quantification based on CD68 marker showed that the scaffold recruited significantly less macrophages compared with the allotransplanted graft, at the same level of the sham group (skin incision only). These results are consistent with our experience with other intrathoracic tissues and organs, such as the aortic root [54] . We therefore suggest the following biocompatibility criteria for decellularized rat oesophagus: (1) absence of MHCI/II-positive cells and (2) ability of cells to adhere and survive on the tissue (indicating the successful removal of cytotoxic decellularization agents). Mechanical strength of the oesophagus is extremely important since it is constantly exposed to stretch and must be distensible but not flaccid. Hence, the engineered scaffold needs to have similar characteristics to the native organ. In order to transport food boluses properly, compliance of the engineered neo-oesophagus must withstand repeated cycles of applied pressure associated with swallowing. Scaffolds that are too weak may rupture or leak, and cause severe conditions such as mediastinitis in the recipient. Conversely, a scaffold that is too stiff could bulge into the trachea and cause dyspnea. We performed several tests to evaluate the mechanical properties of our scaffolds. The distensibility of the oesophagus is vital for allowing food boluses to pass. This parameter is conferred by the structural alterations of the noncontractile matrix proteins (collagen, elastin) of the oesophageal wall, which are responsible for the elastic properties of the organ. As expected, decellularization of the tissue impaired distensibility. However, the distensibility of a reseeded scaffold was almost identical to that of a native organ, suggesting that the reseeding process had positive influences on the scaffolds’ biomechanical properties. A long-term stress test indicated that the scaffold could withstand over 10,000 inflation–deflation cycles over a 72-h period, without any leakage. Our protocol induced a decrease in longitudinal strength compared with native tissue, which is likely due to loss of cell skeletons and a reduction of some ECM proteins. Bhrany et al. [44] presented a decellularization protocol that requires 225.5 h, and reported an ~28% decrease in burst pressure. However, our 3-h protocol yielded an organ with no decrease in burst pressure, suggesting that extended exposure time to reagents is a significant factor contributing to loss of biomechanical strength. We found that after reseeding and culture for 3 weeks, the original longitudinal strength was restored, in a similar manner to the changes in distensibility. Oesophageal tissue regeneration requires blood and nutrient supply, and thus neovascularization [55] . Our decellularization protocol resulted in the retention of the majority of VEGF, and the scaffold was also found to possess strong pro-angiogenic properties as demonstrated by the induction of angiogenesis in a CAM assay. The presence of vasculature could also be detected after the orthotopical transplantation by the presence of von Willebrand factor and muscle-positive vessels. In the present study, we reseeded the graft with adult stromal cells, literally BM-MSCs. We showed that these adherent cells could spontaneously change gene- and protein expression in a tissue-specific manner. The advantage of this cell source, compared with other cell types such as embryonic stem cells, induced pluripotent stem cells or tissue-specific progenitor cells, is the lack of ethical concerns, the ease to obtain and maintain their non-immunogenicity and the great potential for clinical transfer. Notably, we successfully transplanted the reseeded oesophageal scaffold into an orthotopic position and showed patency and normal function over the entire 2-week study period. We chose this period as it represents ~1-year in human life [56] , and we observed most complications in our clinical biological scaffold transplants within 1 year. As a control, we resected and re-anastomosed a 15-mm segment of the cervical oesophagus. Interestingly, we found that the animals receiving the grafts had more favourable weight curves, a finding that could be attributed to the patency resulting from a circumferential segmental replacement of a functional scaffold or the documented immunomodulatory effects of the seeded MSCs [57] . Another possible explanation is that the control autografts potentially were suffering from ischemia in a greater extent, as the original blood supply was damaged surgically. The tissue-engineered grafts, in contrast to the autografts, were repopulated with cells that survived based on only diffusion (as in the incubator). Neither of the groups regained their preoperative weight, but this may be due to the extent of the operation and suboptimal postoperative care compared with that in human operations. In the clinical setting after oesophagectomy, patients are usually given supplemental nutritional support intravenously or via a jejunostomy, and have a nasogastric tube to relieve the anastomoses for 7 days. Despite these measures, severe complications occur in 55–70% of the cases [58] and on average, a weight loss of 13% is seen [59] . We did not find any GFP positive cells in the explanted oesophageal grafts. This is probably attributed to either lack of initial vascularization or cell detachment due to physical stress (swallowing). The harvested grafts showed a mature epithelium and initial regeneration of a muscular layer. The epithelium was found to be a functional microbial barrier in vivo (as demonstrated by TEM images), and the barrier function was also demonstrated in vitro by a biotin assay. The regenerated tissue also showed evidence of neo-neurogenesis and neo-angiogenesis. The two limitations of this study, from a translational point of view, are as follows: (1) the histology of the rodent is different from humans. In fact, the rat has mainly a skeletal muscle composition of the oesophagus, while humans have a skeletal (oral side)—smooth muscle (gastric side) transition. The epithelium is also keratinized in the rat but not in humans. (2) The transplantation of 20% of the oesophageal length might not be clinically useful. We chose to replace the entire cervical oesophagus only as the entire replacement likely would have needed extensive postoperative care such as more extensive and complex pain control, chest drainages, total parenteral nutritional support and so on, which may raise ethical concerns. We are well aware of these limitations, but aimed to evaluate the feasibility of the presented approach first in a small animal model, and feel that the knowledge acquired is encouraging and must be evaluated in a larger animal model where a total replacement may be more feasible In conclusion, we have developed a fast and reproducible perfusion protocol for decellularization of the rat oesophagus, resulting in an ideal biological scaffold with all necessary requirements for a transplantable graft. We have extensively characterized the decellularized scaffold for its biological, structural, mechanical, biocompatibility and angiogenic properties. We further demonstrated the non-immunogenicity of the graft in an immunocompetent small animal model. We successfully reseeded the decellularized scaffold with BM-MSCs, an easily obtained human cell type, and demonstrated spontaneous differentiation of the MSCs towards oesophageal-specific cell types, which in turn suggests the presence of bioactive molecules in our scaffold. This is the first report of successful development and transplantation of a decellularized donor oesophagus, reseeded with allogeneic adult stromal cells that yields a functional graft in vivo with regenerative properties. Ongoing studies are underway to further investigate the cell-to-cell organization and interaction in vivo , and to identify whether the regeneration and/or organ maturation processes observed in our non-acute maturing graft transplant are driven by the seeded cells, migratory cells from the anastomotic site, or neighbouring resident and circulating progenitor and stromal stem cells. Animal care and organ harvesting Animal procedures were approved by the Stockholm South Ethical Committee (numbers 12–13). Ninety-four 8-week-old male Sprague–Dawley rats (Charles River) were used in the study. Animals were euthanized by an intraperitoneal pentobarbiturate overdose (150 mg kg −1 ). The oesophagus was explanted, placed in ice cold Dulbecco’s PBS (Gibco, Life Technologies) containing 1% antiobiotics–antimycotics (Gibco, Life Technologies) and were stored at 4 °C. Decellularization of oesophagus The oesophagus was rinsed in PBS (Gibco, Life Technologies), stripped of connective tissue and cannulated in both ends with plastic catheter 20G I.V. catheters (Terumo). The organs were fixed to the cannulas using 6-0 Prolene ligatures (Ethicon) and were fitted to the perfusion system (Hugo Sachs Elektronik) with a peristaltic pump set to 9 ml min −1 (Ecoline, Ismatec). The protocol consisted of two cycles of 30 min 4% w/w sodium deoxycholate (Sigma-Aldrich) with 2,000 kunitz units DNase-I (Sigma-Aldrich) and 30 min of MilliQ water. The second MilliQ step included 2 mM EDTA (Sigma-Aldrich). Tissues were rinsed for 60 min using PBS (Gibco, Life Technologies). All steps were performed at room temperature, with a reagent volume of 200 ml. Histology and immunohistochemistry Samples were frozen, sectioned at 8 μm, fixed in 4% formalin and stained for H&E (Histolab), Masson’s Trichrome (Sigma-Aldrich) and 4′,6-Diamidino-2-Phenylindole (DAPI; Sigma-Aldrich) were used to evaluate tissue decellularization and morphology. For fluorescence immunohistochemistry, samples were blocked for 60 min in 5% goat serum at room temperature (Invitrogen, Life Technologies) in PBS with 0.3% Triton X (Sigma-Aldrich) and were incubated overnight at 4 °C with primary antibody at the respective concentrations: Laminin (1:100; Abcam Ab11575), Elastin (1:50; Abcam Ab21610), Fibronectin (1:100; Abcam Ab6328), Collagen I 1:100 (Ab34710), Collagen IV (1:100; Abcam Ab6586), MHC I (1:20; AbcamAb22367 FITC-conjugated), MHCII (1:100; Abcam Ab23990), MyoD1 (1:100; Abcam ab16148), Pan-keratin (C11) (1:800; Cell Signaling Technology no. 4545), Gap43 (1:200; Cell Signaling Technology no. 8945), Desmin (1:100; Cell Signaling Technology no. 5332), von Willebrand factor (1:1,600; Abcam Ab6994), beta-III-tubulin (1:200; Covance MMS-435P), VEGF (1:100; Abcam Ab1316), Ki-67 (1:200; Fisher Scientific; SP6), ZO-2 (1:50; Cell Signaling Technology; 2847-S). Sections were washed three times in PBS and secondary antibodies were applied for 1 h at room temperature: Goat-anti-rabbit (1:500; Life Technologies; a11037), Goat-anti-mouse (1:500; Life Technologies; a11032). Sections were washed three times in PBS and mounted with Fluoroshield with DAPI (Sigma-Aldrich). Fluorescent intensity of ECM protein staining were quantified using ImageJ [60] . Micro-CT The CT images of decellularized and native oesophagus were captured using FOV 5 and a 3-min scan time on Quantum FXmCT (Caliper, Perkin Elmer Inc.). SEM and fibre evaluation Samples were fixed in 2.5% glutaraldehyde (Merck) in 0.1 M cacodylate buffer (Prolabo) for 2 h in room temperature, rinsed in cacodylate buffer and dehydrated in ethanol gradient. Samples were dried, gold-sputtered and visualized with SEM (JSM6490, JEOL). The assessment of fibre orientation was based on the image analysis of micrographs from SEM performed by custom-made software (Matlab, The Mathworks, Natick, MA, USA) previously presented [61] . SEM micrograph was first processed to extract a square image. A circular mask is then superimposed before binarization. This condition, allowing analysis of the central region of the image, is necessary in order to prevent the introduction of artifact from the rotation of a square image around its centre from 0° to 360°. This rotation is the next step. The resulting image is binarized, setting a threshold level and then rotated around its centre in increments of 2°. For each direction, the fraction of bright pixels is computed and the resulting s.d. calculated. Results were graphically presented by means of a unitary polar plot, which is representative of the analysed ECM. In order to quantify the investigated pattern, the eccentricity of the ellipse fitting the obtained polar plot was proposed as a measurement index and is defined as follows: where A M is the major semiaxis (the maximum radius of the polar plot) and A m is the minor semiaxis (the 90° value of the polar plot). According to this formulation, E =1 indicates a straight line (unidirectional fibre alignment) and E =0 indicates a perfect circle (randomly arranged fibres). Moreover, the orientation of the fitting ellipse is representative of the average fibre alignment. Magnetic resonance imaging and tractography The ex vivo Diffusion Tensor Imaging (DTI) data were acquired on a 9.4 T MR-scanner (Varian inc, Yarnton). The native and decellularized oesophagi were threaded on a plastic tube to maintain an open lumen. The samples were immersed in Fomblin (SolavaySolexis) in a plastic syringe and placed in a birdcage coil of 16-mm inner diameter. The DTI data were acquired using a spin echo sequence, prepended by a gradient spin echo-sensitive to diffusion. A total echo time of 16.39 ms, tr of 2.1 s and NEX=12 were used. Thirty-two contiguous slices of 0.3-mm thickness were acquired with a matrix size of 256 by 256 covering a field of view of 12.8 by 12.8 mm 2 . Diffusion weighted data from 30 different directions were acquired and complemented by a reference image, where the diffusion-sensing gradients were set to zero. The data were zero-filled to 512 by 512 before Fourier transformation, resulting in a pixel size of 25 by 25 μm. A six-parameter tensor was fitted to each voxel in the DTI data. Probabilistic fibre tracking was performed based on the tensors, employing an angular threshold of 50°. The tracts were then visualized with conventional colour-coding. In order to reduce noise, only tracts longer than 0.3 mm were visualized. The tractography was implemented using the Diffusion Toolkit ( http://trackvis.org/dtk ). CAM assay For evaluation of in vivo angiogenic properties, the chicken embryo CAM assay was performed, in accordance with our previous publication [62] . Briefly, fertilized White Leghorn chicken eggs were incubated at 37 °C with constant humidity for 3 days. A square window was opened in the shell and after the removal of 2–3 ml of albumin, sealed with glass and the egg returned to incubator for 5 more days. Decellularized oesophagus (1 mm 3 ) was then placed on the CAM. For control groups, collagen sponges (Gelfoam Upjohn) containing PBS (negative control) or 200 ng of recombinant VEGF (R&D Systems; positive control) were used [57] . The eggs were incubated for 12 days and photographs and image analysis were carried out (Olympus). On day 12, the angiogenic response was evaluated by an image analyser system as the number of vessels converging towards the implants and the sponges. Samples were then removed from the CAM, washed with PBS, fixed for 24 h in 10% neutral buffered formalin solution (pH 7.4) and treated for SEM observation as above reported. Burst pressure and stress test Two-centimetre segments of native and decellularized oesophagi were attached to 20 G cannula (Terumo) and the opposite end was ligated (Ethicon). The cannula was connected to a syringe pump (PHD2000, Harvard Apparatus) and a pressure transducer (P1500, Hugo Sachs Elektronik). The pump injected air at a rate of 8 ml min −1 and PC-software (Hugo Sachs Elektronik) was used to measure the pressure/volume curve. The stress test was conducted by injecting and withdrawing 800 μl of air. A total of 10,000 cycles were used during 72 h, of which the scaffold was submerged in PBS. Longitudinal mechanical test Longitudinal strength was measured with a universal testing machine (UTM, Lloyd LRX) [27] . The samples were clamped to the UTM grips by means of two strips of emery paper. The force at break and the strain at break, defined as the ratio between the grip displacement and the initial gripping distance, were recorded. Isolated pressurized small organ bioassay Fresh, decellularized and reseeded oesophagi were pulled onto stainless steel cannulas, subsequently secured with 4-0 polyester thread (Ethicon) or stainless steel wire (diameter 0.04 mm) and gently stretched with the vernier. The cannulas were attached to a 10-ml organ tissue bath ( www.livingsys.com ), which was continuously superfused with 37 °C physical salt solution (PSS; composition in mmol l −1 : NaCl 119; KCl 4.7; NaHCO 3 25; KH 2 PO 4 1.2; MgSO 4 1.2; Na 2 EDTA 0.03; D-(+)-glucose 5.5; CaCl 2 2.5) and gassed with 95%O 2 /5%CO 2 at ~10 ml min −1 . After mounting, the lumen was gently perfused with PSS using a pressure servo-controller with a peristaltic pump until a stable intra-luminal pressure of 20 mm Hg was maintained for at least 60 s. Samples not meeting this criterion were not taken for further experimentation. After tissues were equilibrated at a distending intraluminal pressure of 20 mm Hg (30 min), it was stretched transversally by rapidly increasing intraluminal pressure in steps (each lasting 2 min) to 60, 120, 180 and 240 mm Hg. The acquisition of images was performed before the next pressure step for offline diameter analysis with a Dino-Lite USB-microscope ( www.dino-lite.eu ). Each tissue was subjected to a pressure-diameter protocol under ‘resting conditions’ (that is, perfused with PSS with CaCl 2 and in the absence of external stimuli). The diameter of each tissue was measured in triplicates at three random points along the longitudinal axis and the distensibility index was calculated by ( D i / D 20 ) × 100, whereby the D i is the diameter recorded at a certain distending pressure and D 20 is the diameter at a distending pressure of 20 mm Hg. BM-MSC isolation and seeding to scaffold The bone marrow was flushed with PBS (Gibco, Life Technologies) and the cell suspension was centrifuged for 10 min at 300 g . The pellet was re-suspended in culture media: DMEM low glucose, 10% FBS and 1% antibiotic–antimycotic (all from Invitrogen, Life Technologies) and the adherent fraction was cultured to 80% confluency. We characterized the cells using flow cytometry for MSC-specific positive: CD29, CD44, CD59, CD73, CD90, CD106 and negative markers CD11b, CD31 , CD45 (ref. 36 ). To perform the seeding studies, 6-mm discs of the scaffold were dissected with a punch biopsy. Rat MSCs at passage 4 were used and seeded at cell densities of 80,000 cells cm −2 . GFP electroporation Rat MSCs at passage 2 were GFP-labelled by using the pT2-Amaxa-GFP transposon and the SB100X sleeping beauty transposase plasmids. Two microgram pT2/-Amaxa-GFP and 1 μg SB 100 × were transfected into cells using the Neon Electroporation system (Invitrogen, Life Technologies). Cells were sorted for GFP expression using a fluorescent-activated cell sorter (BD). Tubular cell seeding The number of MSCs required for reseeding was calculated by determining the number of cells required to fully cover the surface of the oesophagus based on its surface area and the surface area of the attached cells. Hence, the number of cells N S , required for seeding either the interior or exterior surfaces in order to achieve 100% cell coverage is given by where A a is the average surface area of an attached mesechymal stromal cell (281 μm 2 ). The oesophagus is assumed to be an annular cylinder with diameter (interior or exterior) D s and length L . Typical dimensions of the decellularized oesophagi used in the experiments had interior diameter D i =3.5 mm, exterior diameter D e =4 mm and length L =4 cm. Substituting the given parameter values in the equation gives the number of cells required to seed the interior and exterior surfaces of the oesophagus as N I =1.6 × 10 6 and N O =1.8 × 10 6 , respectively—that is, a total number of ~3.4 million cells. Internal seeding was performed by injecting 600 μl of cell suspension inside the lumen, and both ends were ligated. The scaffold was left in a static condition for 50 min before more media was added. DNA isolation and quantification Uniform full-wall segments (~20 mg) were cut, weighed and DNA extraction was performed according to the manufacturer’s instructions with a DNeasy kit (Qiagen). DNA concentration was measured on a spectrophotometer (Nanodrop, Saveen Werner). Total DNA was normalized to weight to quantify the amount of DNA in samples. Subcutaneous transplantation Adult Sprague–Dawley rats ( n =3 per group) were anaesthetized with subcutaneous injection using a combination of Domitor/Dormicum and Fentanyl (Intervet). Dorsal fur was shaved and a mid-dorsal cutaneous incision was made. A subcutaneous pouch of 1 by 1 cm 2 was bluntly dissected and a 1-cm segment of decellularized or native oesophagus was sutured to the underlying tissue. The negative control was a sham surgery without grafts. The skin was closed with three interrupted sutures (Ethilon). Animals were checked daily and killed on day 5. The transplanted grafts were dissected with a 10-mm margin, frozen in OCT for cryo-sectioning and were stained with H&E. Macrophage staining and visualization A minimum of eight sections per animal ( n =3 per group) were stained for the macrophage marker CD68. Eight-micrometre sections were used. Samples were fixed in 4% formaldehyde for 10 min, and then blocked 1 h at room temperature with Tris-buffered saline and 10% goat serum (Vector Labs, S-1000). Primary antibody CD68 (1:800; Abcam 31630) was incubated overnight in a buffer containing TBS 0.1%, Triton X-100 and 10% goat serum. Secondary antibody (Alexa Fluor 594, Life Technologies, A-11005) and nuclear stain Hoechst (2 μg ml −1 ) were co-incubated for 1 h at room temperature in TBS 0.1% and Triton X-100. All slides were mounted with Vectashield (Vector Labs). For each section, three photographs were taken using a × 25 magnification and the number of macrophages was quantified. The number presented is an average of macrophage cells per section. Real-time quantitative polymerase chain reaction MSCs grown on scaffold and standard cultures were collected for gene expression analysis. RNA extraction was performed with RNeasy mini kit (Qiagen) and RNase free DNase kit (Qiagen) to remove genomic DNA. High-capacity cDNA Reverse Transcription kit (Applied Biosystems) was used to synthesize cDNA. The taqman probes used were: GAPDH (Rn01775763_g1), CD90 (Rn00562048_m1), Desmin (Rn00574732_m1), SP1 (Rn00561953_m1), Myf6 (Rn01503350_g1), Myog (Rn01490689_g1), Krt10 (Rn02350069_m1), Krt14 (Rn01467684_m1) and Krt5 (Rn01533116_g1). The samples were analysed on 7500 Fast Real-Time PCR System (Applied Biosystems). The expression levels for each sample were normalized to GAPDH and relative expression was calculated using the ΔΔ C t method. Results were presented as relative fold change compared with cells grown under standard cultures. Determination of intracellular calcium levels Cells growing on plastic or on 25-μm thick cryosections of decellularized scaffolds were loaded with the 5 μM of Ca2+-sensitive fluorescence indicator Fluo-3/AM (Invitrogen) in cell culture medium at 37 °C for 30 min. Measurements were performed at 37 °C in a heat-controlled perfusion chamber with a cooled back-illuminated EMCCD camera mounted on an inverted microscope equipped with a 25 × /0.8 NA water objective. Excitation at 495 nm was carried out using a Lambda LS xenon-arc lamp equipped with a SmartShutter. Emission wavelengths were detected at 510 nm. KCl was bath-applied at a final concentration of 45 mM. Electrical resistance measurements Electrical resistance through the scaffold was measured using EVOM2 (World Precision Instruments). A custom-made construct was created to mount the epithelium as follows ( Fig. 9d ): a 3-mm hole was made in the middle of a 35-mm petridish. The petridish was placed on four stainless steel distances in a 100-mm dish and was covered with 75 ml PBS (Gibco). Decellularized or reseeded tissue was placed over the 3-mm hole, and a metal ring was used to pull the tissue down. The EVOM2 device was used to measure the resistance over the tissue. Orthotopic transplantation Adult Sprague–Dawley rats ( n =10) were anaesthetized with subcutaneous injection of Domitor/Dormicum and Fentanyl (Intervet). A 3-cm anterior midline, cervical incision was made to reach the trachea that was cut transversally to facilitate breathing. The oesophagus was bluntly dissected and mobilized. A 15-mm section of the oesophagus was resected and replaced with a reseeded, decellularized scaffold. The anastomoses were made with single sutures (7-0 polyprolene, Ethicon), knots outside of the lumen. The muscular layer was closed with continuous suture 6-0 polyprolene (Ethicon) and the skin was closed using interrupted sutures of Ethilon 4-0 (Ethicon). Animals were given liquid food for 7 days, followed by soft diet (Gelfood 76a, Clear H 2 O) until the study end point of 14 days. Pain and general health assessment scales Postoperatively, animals were carefully observed at 2, 12, 24 and every 24 h thereafter. A pain assessment scale [38] that evaluates changes in the animals’ face was used. The scale has four categories including orbital tightening, nose/cheek flattening, ear changes and whisker changes. Each category is judged as absent, moderate or obvious. The Karolinska Institutet health assessment checklist includes six additional categories: general condition, porphyrin staining, movements and posture, piloerection, respiration and skin. Transmission electron microscopy The explanted graft was fixed at room temperature for 30 min in 2% glutaraldehyde (Merck) and 1% paraformaldehyde (Histolab.se) in 0.1 M phosphate buffer, pH 7.4. Samples were rinsed in 0.1 M phosphate buffer, pH 7.4 and post-fixed in 2% osmium tetroxide, 0.1 M phosphate buffer pH 7.4 at 4 °C for 2 h, dehydrated in ethanol followed by acetone and embedded in LX-112 (Ladd). Semi-thin sections were stained with toluidine blue O (Sigma-Aldrich) and used for light microscopy analysis. Ultra-thin sections (~40–50 nm) were cut with a Leica EM UC 6 and contrasted with uranyl acetate followed by lead citrate and were examined in a Tecnai 12 Spirit Bio TWIN transmission electron microscope (FEI company) at 100 kV. Digital images were taken with a Veleta camera (Olympus Soft Imaging Solutions). Biotin assay Biotin assay was performed to functionally evaluate the epithelium as previously described [41] . Briefly, Biotin (Long Arm) NHS (BioNordika) was reconstituted to 1 mg ml −1 and applied to the epithelium for 1 min. Biotin does not penetrate a healthy epithelium due to its crosslinking epithelium. The tissue was then washed 3 × 5 min in PBS, frozen in OCT, sectioned and stained according to the immunohistochemistry section. The secondary antibody used was DyLight 594 Streptavidin (1:500, Bionordika) [58] , [59] , [60] , [61] , [62] . Statistical analysis Results were expressed as mean±s.d. GraphPad Prism 5 (GraphPad Software, USA) was used for statistical analyses. All data was analysed with ANOVA or Student’s t -test. The level of significance was indicated as follow: * P ≤0.05, ** P ≤0.01 or *** P ≤0.001. How to cite this article: Sjöqvist, S. et al. Experimental orthotopic transplantation of a tissue-engineered oesophagus in rats. Nat. Commun. 5:3562 doi: 10.1038/ncomms4562 (2014).